Micro-trace fossils reveal pervasive reworking of Pliocene sapropels by low-oxygen-adapted benthic meiofauna Animal burrowers leave an indelible signature on the sedimentary record in most marine environments, with the seeming exception of low-oxygen environments. In modern sedimentary settings, however, sub-millimetre-sized benthic animals (meiofauna) are adapted to low oxygen and even sulfidic conditions. Almost nothing is known about their impact on ancient marine sediments because they leave few recognizable traces. Here we show, in classic Pliocene-aged anoxic facies from the Mediterranean, the first reported trace fossil evidence of meiofaunal activity and its relation to changing oxygenation. A novel approach utilizing electron imaging of ion-polished samples shows that meiofauna pervasively reworked sediment under oxygen-depleted conditions that excluded macrofauna, fragmenting organic laminae and emplacing 15- to 70-μm-diameter faecal pellets without macroscopically influencing the fabric. The extent of reworking raises the question: how pervasively altered are other sediments presently assumed to lack animal influence and how far into the geological record does this influence extend? The dynamic interaction between marine sediments and burrowing fauna represents one of the key biogeochemical processes on the Earth [1] , [2] , [3] , [4] . Benthic animals facilitate sediment irrigation and oxygen ingress through burrowing [1] , [2] , [3] and accelerate organic matter (OM) degradation through ingestion, physical comminution and enzymatic breakdown [1] , [5] , [6] . Since their proliferation in the Cambrian, animal burrowers have left an indelible signature on the sedimentary record in almost all marine environments [7] , with the seeming exception being low-oxygen environments that are typified by laminated sediments lacking visible evidence of animal activity [8] . In modern environments, however, sub-millimetre benthic (meiofaunal) animals are adapted to and prosper under low-oxygen, even sulfidic conditions [9] , [10] , [11] . Although less well known than the larger benthic fauna, meiofauna (44 to 500 μm in size [10] ) are more abundant in most modern marine sediments [10] and occupy a greater range of environments, including oxygen-depleted environments [9] , [11] , [12] , [13] . Although they navigate around sand grains, they ingest the finest, most chemically reactive sediment fraction [10] and have an impact on sediment biogeochemistry similar to the macrofauna. For example, meiofaunal burrowing stimulates the decomposition of sediment OM [14] , [15] , [16] , increases microbial growth [17] and produces a dense net of fine burrows [18] , [19] that increase solute transport between 1.7- and 3.6-fold relative to molecular diffusion [16] , [20] , [21] , increase sulfide oxidation [10] and shorten pore-water turnover to only 1–3 years [18] . Adaptations, such as reduced size, small cross-section allowing efficient oxygen diffusion and navigation between large grains, high sulfide tolerance and low metabolic needs for oxygen, allow certain meiofauna to prosper where macrofauna do not [10] . Although they are ubiquitous in modern settings, almost nothing is known about the impact of meiofauna on biogeochemical cycling in the past because understanding of ancient (soft-bodied) benthic animal activity comes almost exclusively from traces rather than body fossils [22] . In contrast to benthic macrofauna, which produce macroscopically visible trace fossils and leave clear evidence of bioturbation [22] , the record of meiofaunal activity in ancient marine sediments is cryptic and all but unknown [10] , [22] , [23] , with some inferences drawn from experiments and modern sediments [12] , [22] , [24] , [25] . Although the fossil record cannot currently be used to support any general hypothesis about the timing and impact of meiofaunal animal evolution [26] , it has been proposed that meiofauna may significantly predate the advent of larger motile animals [25] , [27] . Here we show, in anoxic, Pliocene-aged sapropels from the Mediterranean (Ocean Drilling Program Site 969), the first reported trace-fossil evidence of meiofaunal activity and its relation to changing oxygenation. The Pliocene sapropels are a classic low-oxygen facies commonly used as an analogue system for the widespread, organic carbon-rich black shales that characterize economically and oceanographically important intervals in the Palaeozoic and Mesozoic [28] , [29] . We image compositional differences using backscatter electron (BSE) microscopy of ion polished samples to demonstrate that meiofauna pre-dated macrofaunal burrowing, providing a leading edge of irrigation and pelletization in low-oxygen sediments. As in modern low-oxygen environments, meiofauna pervasively ingested the clay-size fraction while showing very limited influence on sediment fabric by not mixing sediment vertically or disrupting visible grains. The cryptic nature of this type of bioturbation may mean that animal influence on sediments occurred in a wider range of paleoenvironmental settings than previously appreciated. Depositional setting and origin of lamination Cyclical deposition of interbedded organic-rich sapropels and organic-lean marls in the eastern Mediterranean has been linked to orbital forcing of the African monsoon [30] , [31] , [32] , with water-column stratification and inhibited deep-water renewal contributing to OM enrichment in sapropel intervals [32] , [33] . Sediment lamination, elevated concentrations of redox-sensitive trace elements [28] , an abundance of framboidal pyrite [34] and the presence of isorenieretane [35] , a biomarker characteristic of photosynthetic green sulphur bacteria, indicate that the ODP Site 969 Pliocene sapropels investigated here were deposited under anoxic and periodically sulfidic conditions. BSE imaging shows that OM in the lower-most part of the sapropels occurs mainly as 5–15 μm organoclay aggregates and grains. As total organic carbon (TOC) content increases towards the sapropel centre, it is increasingly concentrated in discrete OM laminae ( Figs 1 and 2 -B4), separated by OM-lean laminae composed mainly of detrital silicates (silt+clay), with abundant framboidal pyrite throughout. Sediment carbonate content, mainly plankton microfossils (coccoliths and foraminifera), decreases as TOC and sediment lamination increase, reflecting a switch from calcareous plankton typical of marl deposition to productivity dominated by siliceous plankton during sapropel deposition [36] . The discrete nature and moderate lateral continuity of the OM laminae (0.1–5 mm), their thickness (up to 60 μm) and the paucity of detrital grains ( Fig. 3d ) within them is consistent with episodic OM delivery through seasonal mass sedimentation of mat-forming diatoms [37] , [38] and more continuous, year-round (hemi)pelagic sedimentation of mineral detritus. The siliceous diatom tests subsequently dissolve because of silica undersaturation prevalent in the Mediterranean [37] , leaving behind laminae composed largely of OM. 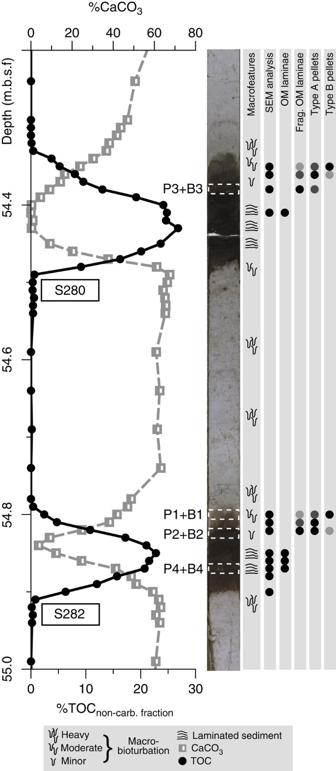Figure 1: Summary of bulk sediment properties and microfabrics in two Pliocene sapropels. Per cent TOC of the non-carbonate fraction (black circles) and per cent CaCO3(grey squares) in two Pliocene sapropel cycles from ODP Site 969, plotted against depth (metres below sea floor (m.b.s.f.)). Site 969 is located on a regional high on the Mediterranean Ridge in 2,200 m water depth41, approximately 100 km south of the island of Crete. The sampled interval (Hole A, Core 6H, Section 6, 125 cm to Section 7, 60 cm) corresponds to sapropels i280 and i282 (ref.31). Dashed white rectangles on the core photo mark the location of samples presented inFig. 2. Also shown are the macroscopic sediment fabric (bioturbated versus laminated), sampling locations of all sediments analysed by scanning electron microscope BSE imaging, the occurrence of intact OM laminae, fragmented OM laminae (frag. OM laminae) as well as Type A (nematode) and Type B (polychaete) faecal pellets. Black to light grey marker colour indicates decreasing abundance. Figure 1: Summary of bulk sediment properties and microfabrics in two Pliocene sapropels. Per cent TOC of the non-carbonate fraction (black circles) and per cent CaCO 3 (grey squares) in two Pliocene sapropel cycles from ODP Site 969, plotted against depth (metres below sea floor (m.b.s.f.)). Site 969 is located on a regional high on the Mediterranean Ridge in 2,200 m water depth [41] , approximately 100 km south of the island of Crete. The sampled interval (Hole A, Core 6H, Section 6, 125 cm to Section 7, 60 cm) corresponds to sapropels i280 and i282 (ref. 31 ). Dashed white rectangles on the core photo mark the location of samples presented in Fig. 2 . Also shown are the macroscopic sediment fabric (bioturbated versus laminated), sampling locations of all sediments analysed by scanning electron microscope BSE imaging, the occurrence of intact OM laminae, fragmented OM laminae (frag. OM laminae) as well as Type A (nematode) and Type B (polychaete) faecal pellets. Black to light grey marker colour indicates decreasing abundance. 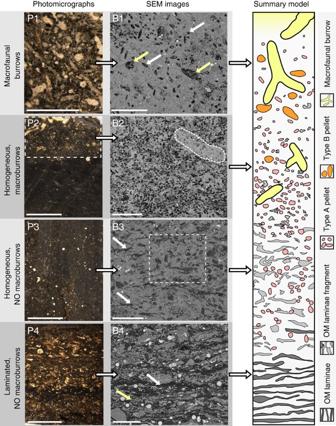Figure 2: Summary model showing evolution of sapropel fabric with meiofaunal bioturbation. Photomicrographs and BSE images of sample intervals outlined inFig. 1showing progression from laminated sapropel (P4+B4), partially laminated to homogeneous meiofaunally bioturbated (P3+B3) and finally meiofaunally and macrofaunally bioturbated sediment (P1 and B1), with summary model. (P4) Photomicrograph of S282, laminated sapropel centre (54.87 metres below sea floor (m.b.s.f.)). Scale bar is 3 mm. (B4) Example of strongly laminated sapropel (S282, 54.85 m.b.s.f.) with alternating OM laminae (white arrow) and organic-poor detrital laminae (yellow arrow). Note the absence of faecal pellets and OM laminae fragments. Scale bar is 40 μm. (P3) Macroscopically partially laminated to homogeneous transitional zone (54.36 m.b.s.f.) between macroscopically burrowed (Chondrites) and laminated intervals in S280. No macroscopic evidence of bioturbation. (B3) Although no macroscopic trace fossils were observed (P3), BSE imaging of this sample shows comprehensive reworking by meiofauna (see alsoFig. 4), identifying <300-μm-long fragments of formerly more continuous OM-rich laminae (examples marked by white arrows). These have been physically disrupted by meiofaunal burrowing but have not been ingested. Note also abundance of type A, OC-rich faecal pellets. Scale bar is 150 μm. (P2) Transition from moderately bioturbated to homogeneous intervals in S282 (54.82 m.b.s.f.). Scale bar is 3 mm.Chondritestrace fossils are concentrated in the upper third of the image (outlined), the subsection subsequently analysed by scanning electron microscope. (B2) BSE image of S282 (54.82 m.b.s.f.) showing high abundance of type A meiofaunal, OC-rich faecal pellets. Note well-preservedChondritestrace fossil (dashed outlined) overprinted on earlier meiofaunal traces. Scale bar is 250 μm. (P1) Photomicrograph of heavily burrowed uppermost S282, ODP Site 969 (54.80 m.b.s.f.). Scale bar is 3 mm. OverlappingChondritesmacrofaunal trace fossils are infilled with light-coloured, carbonate-rich material derived from overlying marl. (B1) BSEI of the same sample shows that OM (dark grey) is concentrated in two benthic meiofaunal faecal pellet morphotypes. Morphotype A: 15–35 μm ovoid (white arrow) and 30–70 μm elongate (white arrow); Morphotype B: 100–300 μm elongate (yellow arrow) and 60–100 μm circular to oval (yellow arrow). Scale bar is 250 μm. Full size image Figure 2: Summary model showing evolution of sapropel fabric with meiofaunal bioturbation. Photomicrographs and BSE images of sample intervals outlined in Fig. 1 showing progression from laminated sapropel (P4+B4), partially laminated to homogeneous meiofaunally bioturbated (P3+B3) and finally meiofaunally and macrofaunally bioturbated sediment (P1 and B1), with summary model. (P4) Photomicrograph of S282, laminated sapropel centre (54.87 metres below sea floor (m.b.s.f.)). Scale bar is 3 mm. (B4) Example of strongly laminated sapropel (S282, 54.85 m.b.s.f.) with alternating OM laminae (white arrow) and organic-poor detrital laminae (yellow arrow). Note the absence of faecal pellets and OM laminae fragments. Scale bar is 40 μm. (P3) Macroscopically partially laminated to homogeneous transitional zone (54.36 m.b.s.f.) between macroscopically burrowed ( Chondrites ) and laminated intervals in S280. No macroscopic evidence of bioturbation. (B3) Although no macroscopic trace fossils were observed (P3), BSE imaging of this sample shows comprehensive reworking by meiofauna (see also Fig. 4 ), identifying <300-μm-long fragments of formerly more continuous OM-rich laminae (examples marked by white arrows). These have been physically disrupted by meiofaunal burrowing but have not been ingested. Note also abundance of type A, OC-rich faecal pellets. Scale bar is 150 μm. (P2) Transition from moderately bioturbated to homogeneous intervals in S282 (54.82 m.b.s.f.). Scale bar is 3 mm. Chondrites trace fossils are concentrated in the upper third of the image (outlined), the subsection subsequently analysed by scanning electron microscope. (B2) BSE image of S282 (54.82 m.b.s.f.) showing high abundance of type A meiofaunal, OC-rich faecal pellets. Note well-preserved Chondrites trace fossil (dashed outlined) overprinted on earlier meiofaunal traces. Scale bar is 250 μm. (P1) Photomicrograph of heavily burrowed uppermost S282, ODP Site 969 (54.80 m.b.s.f.). Scale bar is 3 mm. Overlapping Chondrites macrofaunal trace fossils are infilled with light-coloured, carbonate-rich material derived from overlying marl. (B1) BSEI of the same sample shows that OM (dark grey) is concentrated in two benthic meiofaunal faecal pellet morphotypes. Morphotype A: 15–35 μm ovoid (white arrow) and 30–70 μm elongate (white arrow); Morphotype B: 100–300 μm elongate (yellow arrow) and 60–100 μm circular to oval (yellow arrow). Scale bar is 250 μm. 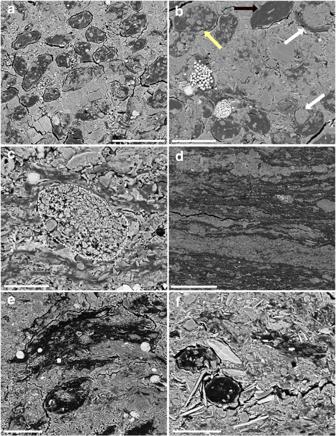Figure 3: Scanning electron microscope images of laminated and meiofaunally burrowed sapropel intervals. (a) Close-up view of the transitional interval (54.82 metres below sea floor (m.b.s.f.)) between the moderately macrobioturbated and homogeneous S282 intervals shown inFig. 2P2+B2. Note the concentration of OM in an abundance of OC-rich, Type A meiofaunal faecal pellets. Scale bar is 40 μm. (b) OM-rich, type A faecal pellets in upper, bioturbated S282 (54.82 m.b.s.f.). Faecal pellets contain variable quantities of inorganic material similar to that of the mineral matrix, with faecal pellets ranging from mainly organic (black arrow) to mixed mineral-organic composition (yellow arrow). White arrows show OM-rich faecal pellets overprinted by smaller, OM-poor faecal pellets or burrow infill, derived from inorganic mineral matrix. Scale bar is 25 μm. (c) Planktonic faecal pellets (white outline) within the laminated interval of S282 (54.87 m.b.s.f.). These rare pellets are not associated with disruption of the sediment lamination and, unlike the OM-rich pellets within the bioturbated interval, they are porous and compositionally distinct from the mineral matrix, consisting mainly of skeletal fragments of calcareous plankton. Deformation of OM laminae around these pellets demonstrates their early origin, before compaction of the sediment, again consistent with a pelagic origin. Scale bar is 15 μm. (d) Strongly laminated sapropel (S280, 54.41 m.b.s.f.) with alternating discrete OM and organic-poor detrital laminae. Scale bar is 75 μm. (e) Type A meiofaunal faecal pellet with OM laminae fragment in S280 from ODP Site 967 (Site 967, Hole B, Core 9, Section 6, 14–15 cm). Scale bar is 25 μm. (f) Two type A meiofaunal faecal pellets with OM laminae fragments in S282 from ODP Site 964 (Site 964, Hole A, Core 9, Section 5, 89–90 cm). Scale bar is 20 μm. Full size image Figure 3: Scanning electron microscope images of laminated and meiofaunally burrowed sapropel intervals. ( a ) Close-up view of the transitional interval (54.82 metres below sea floor (m.b.s.f.)) between the moderately macrobioturbated and homogeneous S282 intervals shown in Fig. 2 P2+B2. Note the concentration of OM in an abundance of OC-rich, Type A meiofaunal faecal pellets. Scale bar is 40 μm. ( b ) OM-rich, type A faecal pellets in upper, bioturbated S282 (54.82 m.b.s.f.). Faecal pellets contain variable quantities of inorganic material similar to that of the mineral matrix, with faecal pellets ranging from mainly organic (black arrow) to mixed mineral-organic composition (yellow arrow). White arrows show OM-rich faecal pellets overprinted by smaller, OM-poor faecal pellets or burrow infill, derived from inorganic mineral matrix. Scale bar is 25 μm. ( c ) Planktonic faecal pellets (white outline) within the laminated interval of S282 (54.87 m.b.s.f.). These rare pellets are not associated with disruption of the sediment lamination and, unlike the OM-rich pellets within the bioturbated interval, they are porous and compositionally distinct from the mineral matrix, consisting mainly of skeletal fragments of calcareous plankton. Deformation of OM laminae around these pellets demonstrates their early origin, before compaction of the sediment, again consistent with a pelagic origin. Scale bar is 15 μm. ( d ) Strongly laminated sapropel (S280, 54.41 m.b.s.f.) with alternating discrete OM and organic-poor detrital laminae. Scale bar is 75 μm. ( e ) Type A meiofaunal faecal pellet with OM laminae fragment in S280 from ODP Site 967 (Site 967, Hole B, Core 9, Section 6, 14–15 cm). Scale bar is 25 μm. ( f ) Two type A meiofaunal faecal pellets with OM laminae fragments in S282 from ODP Site 964 (Site 964, Hole A, Core 9, Section 5, 89–90 cm). Scale bar is 20 μm. Full size image Identified faecal pellet classes OM-rich faecal pellets, which we interpret to be primarily of benthic meiofaunal origin (see below), are present throughout the upper 3–4 cm of S282 and S280 ( Figs 1 and 2 ) but decrease in abundance towards the upper sapropel–marl interface. Two distinct OM-rich pellet morphotypes can be identified in cross-section. Morphotype A, oval to elongate 30–70 μm pellets (length/width ratios of 2–4), are present throughout the bioturbated intervals of both S282 and S280 ( Figs 1 and 2 ). These occur together with circular to ovoid 15–35 μm pellets (length/width ratios of 1–2), which are more likely to be type A pellets imaged across their long axes than a distinct morphotype ( Fig. 3a ). Morphotype B are larger (100–300 μm) oval pellets (length/width ratio ≈2) that are mainly restricted to the top 1 cm of both S282 and S280 ( Figs 1 and 2 ), although they occur infrequently at greater depths. These, again, occur together with smaller circular to oval pellets (60–100 μm diameter), representing type B pellets imaged across their long axes. Superimposed on the pelletized fabric are Chondrites trace fossils that, unlike the faecal pellets, are readily identified by visual inspection. We interpret these macrobenthic trace fossils to be later modifications to the sediment by downwards burrowing organisms because they are infilled with lighter-coloured, carbonate-rich material derived from the overlying marl and have well preserved, sharp outlines with no evidence of meiofaunal reworking ( Fig. 2 ). Chondrites trace fossils are most abundant in the overlying marl and top 1 cm of each sapropel, but can extend 2–3 cm downwards into the sapropel. Importantly, BSE imaging of S280 identifies a macroscopically partially laminated to homogeneous transitional zone situated between the laminated interval and the pelletized and macroscopically burrowed ( Chondrites ) interval. This homogeneous zone is characterized by fragmentation and deformation of OM laminae, and partial pelletization of the sediment ( Fig. 2 -B3), but does not show macrofaunal burrowing traces ( Fig. 2 -P3). A benthic origin for type A and type B faecal pellets Assessing the palaeoenvironmental significance of faecal pellets is dependent on distinguishing their planktonic or benthic origin. In general, benthic pellets are ovoid in shape and densely packed [39] . Silt grains in pellets are smaller than in the surrounding sediment due to size exclusion during ingestion, but the inorganic mineral components of the pellets are similar to the surrounding mineral matrix [39] . Finally, pellets of benthic origin are commonly associated with disrupted sedimentary layering [40] , whereas planktonic pellets are sedimentary grains within layering and so are not associated with disruption of the sediment fabric. Planktonic pellets are commonly cylindrical with tapered ends, porous or loosely packed and generally contain a high percentage of biogenic debris and intact tests, pigments and organic materials [39] . Unlike benthic pellets, planktonic pellets are commonly compositionally and texturally distinct from the sediment matrix [39] , [40] . We interpret both OM-rich pellet morphotypes A and B to be of benthic origin, whereas the rare, OM-poor, porous pellets that were observed only in laminated intervals are likely of planktonic origin ( Fig. 3c ). The small size and excellent preservation of the type A faecal pellets makes a planktonic origin unlikely [39] . Estimated settling times ranging from 26 to 58 days (Stokes’ Law: 45 μm diameter spherical particle, volumetrically equivalent to largest type A pellets; Site 969 water depths of 2,200 m (ref. 41 ); 40–80 vol.% OM with density=1.2 g cm −3 ; 60–20 vol.% inorganic mineral material with density=2.65 g cm −3 ; 17 °C water temperature; 39 PSU, practical salinity units) are sufficiently long for significant physical and chemical degradation of these pellets to occur, and would not produce a concentrated interval of pellets as they would be swept around the basin by currents. Both type A and type B pellets are OM-rich, have a densely packed texture and show no evidence of burial compaction, consistent with compaction and dewatering of pellets within benthic infaunal guts preceding general sediment dewatering and compaction. The pellets show a compositional continuum ( Figs 3b and 4e,f ) ranging from OM-rich pellets largely free of inorganic material to relatively OM-lean, mineral-rich pellets. Although excluding larger silt grains, the inorganic mineral component within the faecal pellets is compositionally and texturally similar to the sediment in adjacent laminae. These observations are consistent with variable mixing of interlaminated OM-rich and OM-poor material during selective deposit feeding by benthic meiofauna, but not with a planktonic origin. Most significantly, OM-rich faecal pellets consistently occur in association with fragments of OM-rich laminae ( Fig. 4 ) indicating that physical disruption and fragmentation of OM laminae was caused by the organisms which produced the faecal pellets directly inline or adjacent to disrupted laminae. In situ pelletization is apparent from (i) laminae fragments that are frequently deformed and vertically oriented relative to bedding in arrangements that are consistent with soft sediment deformation but not with sedimentation of OM fragmented in the water column ( Fig. 4a,b ), (ii) meiofaunal burrows or faecal pellets cutting across laminae fragments ( Fig. 4b–e ) and (iii) the progressive up-section decrease in size and abundance of OM laminae fragments coinciding with the greater relative abundance of OM-rich faecal pellets (compare Fig. 2 B1 to B4), which likely reflects more intense meiofaunal burrowing. 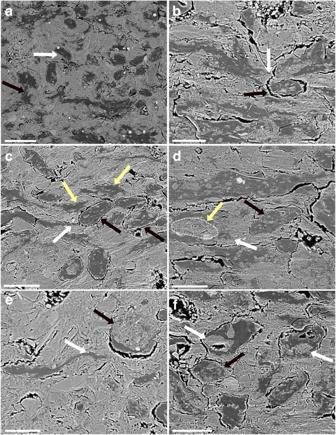Figure 4: Scanning electron microscope images showing benthic origin of meiofauna faecal pellets. All images are of the macroscopically partially laminated to homogeneous zone lacking macrofaunal traces identified inFig. 2(54.36 metres below sea floor (m.b.s.f.)). (a) Faecal pellets (white arrow) intermingled with fragments of OM laminae. The disrupted appearance of laminae fragments, and the vertical orientation relative to bedding of some fragments (black arrow) is indicative of post-depositional, biotic, soft-sediment deformation rather than sedimentation of OM fragmented in the water column. Enlarged fromFig. 2B3. Scale bar is 50 μm. (b) Deformed and fragmented OM laminae (white arrows), with faecal pellet (black arrow) emplaced in the fragmentation zone, suggesting that the organism that produced the faecal pellet also disrupted the OM laminae. Scale bar is 20 μm. (c) Faecal pellets (black arrows) cutting across OM laminae (white arrow). Note also adjacent, deformed OM laminae fragments (yellow arrows), attributed to meiofaunal bioturbation. Scale bar is 40 μm. (d) OM-poor faecal pellet (yellow arrow) cutting across OM laminae fragment. OM-poor pellet is similar in size and shape to an adjacent OM-rich faecal pellet (black arrow). Scale bar is 30 μm. (e) Laminae fragment (white arrow) with adjacent faecal pellet (black arrow) incorporating an OM laminae fragment and inorganic material derived from the surrounding mineral matrix. Scale bar is 20 μm. (f) Faecal pellets with a broad compositional spectrum, showing a range from high (black arrow) to low (white arrow) organic/mineral component ratios. Note also the inclusion of OM-free domains in faecal pellets, composed of material derived from the surrounding mineral matrix. Scale bar is 30 μm. Figure 4: Scanning electron microscope images showing benthic origin of meiofauna faecal pellets. All images are of the macroscopically partially laminated to homogeneous zone lacking macrofaunal traces identified in Fig. 2 (54.36 metres below sea floor (m.b.s.f.)). ( a ) Faecal pellets (white arrow) intermingled with fragments of OM laminae. The disrupted appearance of laminae fragments, and the vertical orientation relative to bedding of some fragments (black arrow) is indicative of post-depositional, biotic, soft-sediment deformation rather than sedimentation of OM fragmented in the water column. Enlarged from Fig. 2 B3. Scale bar is 50 μm. ( b ) Deformed and fragmented OM laminae (white arrows), with faecal pellet (black arrow) emplaced in the fragmentation zone, suggesting that the organism that produced the faecal pellet also disrupted the OM laminae. Scale bar is 20 μm. ( c ) Faecal pellets (black arrows) cutting across OM laminae (white arrow). Note also adjacent, deformed OM laminae fragments (yellow arrows), attributed to meiofaunal bioturbation. Scale bar is 40 μm. ( d ) OM-poor faecal pellet (yellow arrow) cutting across OM laminae fragment. OM-poor pellet is similar in size and shape to an adjacent OM-rich faecal pellet (black arrow). Scale bar is 30 μm. ( e ) Laminae fragment (white arrow) with adjacent faecal pellet (black arrow) incorporating an OM laminae fragment and inorganic material derived from the surrounding mineral matrix. Scale bar is 20 μm. ( f ) Faecal pellets with a broad compositional spectrum, showing a range from high (black arrow) to low (white arrow) organic/mineral component ratios. Note also the inclusion of OM-free domains in faecal pellets, composed of material derived from the surrounding mineral matrix. Scale bar is 30 μm. Full size image The uniform size and appearance of each faecal pellet morphotype is consistent with production by a single organism type. Although the organisms cannot be identified directly, likely candidates can be determined by comparison to the faunal assemblages of modern low-oxygen sedimentary settings [42] . Although the diversity and abundance of benthic macrofauna is severely restricted in environments with dissolved oxygen levels <0.2 ml l −1 , small, surface deposit-feeding polychaetes and their faecal pellets (150–800 μm long) are present in modern sediments deposited under severely dysoxic (0.2–0.1 ml l −1 ) conditions [39] , [40] , [42] , [43] , [44] . The size and ovoid shape of the type B faecal pellets is thus consistent with a small macrofaunal or large meiofaunal polychaete origin [39] . The OM-rich type A pellets, on the other hand, are almost an order of magnitude smaller than those benthic faecal pellets previously described in the geological literature, for example, see refs 39 , 40 , and are too small to be products of benthic macrofauna. Alternatively, benthic meiofauna are ubiquitous in modern marine sediments and are associated with faecal pellets of this size. Benthic copepods, including species of meiofaunal size, are widespread and prolific producers of faecal pellets [10] . However, copepod pellets are typically larger and more elongate than the type A pellets and copepods are rare in severely oxygen-depleted environments [10] , [42] . Other benthic meiofauna belonging to the ‘thiobios’, and characteristic of environments in which hydrogen sulphide and other reduced substances are dominating ecological factors [10] , are adapted to the oxygen-depleted, sulfidic conditions typical of sapropel deposition. The metazoan, meiofaunal ‘thiobios’ includes species within the phyla Platyhelminthes, Gnathostomulida and Gastrotricha, but the morphology, size, absence of a complete gut and/or preference for shallower waters makes these organisms unlikely candidates [10] . However, sulfide-adapted nematodes are widespread members of the ‘thiobios’. Their small size has contributed to a lack of studies of nematode pellet formation but, given that nematodes can ingest fine-grained sediment and OM and occur in deep-water settings [10] , they are likely producers of the type A pellets. Benthic nematodes are a common, widespread class of meiofauna and are particularly dominant in low-oxygen settings because they are able to tolerate severely dysoxic and even sulfidic conditions [10] , [12] , [13] , [45] . A modern meiofauna dominated by nematodes (~ 99% of meiofaunal diversity) occurs under oxygen-depleted, highly sulfidic conditions in Black Sea sediments and within the oxygen-minimum zone off the coast of Chile and Peru [9] , [10] , [11] . Similarly, in the severely dysoxic surficial sediments (0–5 cm) of the modern Santa Barbara Basin, nematodes represent 80–99% of all metazoans [12] . Although marine nematodes have a broad breadth range (8–200 μm cross-sectional diameter), nematodes with a more slender morphology are common in lower-oxygen environments [45] . The nematodes of the Santa Barbara Basin, for instance, have diameters of 50–75 μm (ref. 12 ), closely corresponding to the size range of the type A faecal pellets identified within the sapropels. Although adapted to severely dysoxic and sulfidic conditions, nematodes are not true anaerobes [13] , so that we interpret the concentration of type A pellets to be the product of marine nematodes living in and reworking the sediment during freshening phases of sapropel deposition. Disruption of lamination and concentration of faecal pellets within specific horizons is commonly interpreted to reflect transient increases in bottom-water oxygen levels allowing restricted benthic activity [40] . The gradually decreasing preservation of sediment fabric and lamination up-section from peak sapropel TOC, beginning with fragmentation of discrete OM laminae ( Fig. 2 ) and followed by increasing ingestion and pelletization of OM, likely records a transition from anoxic/sulfidic conditions to merely severely dysoxic conditions capable of supporting benthic nematodes (Type A) and, subsequently, polychaetes (Type B pellets). More oxygenated conditions after marl deposition resumed then provided the conditions required for recolonization by benthic macrofauna, which burrowed downwards forming the Chondrites trace fossils. Thus, both the first appearance of the faecal pellets and the later emplacement of Chondrites fossils record passing of environmental thresholds, that is, increased oxygen or decreased hydrogen sulphide concentrations. Two scenarios can explain the vertical gradient between fully laminated sediment at the sapropel centre and almost complete pelletization of the uppermost sapropel. In the first scenario, meiofaunal nematodes are present within the sediment well before the low-oxygen-adapted polychaetes, and pelletization of the sediment is mainly syndepositional. Alternatively, the pelletization of the sediment postdates deposition of the sapropel. Here, the burrowing and pelletization gradient results from the higher tolerance of the nematodes to anoxic, sulfidic conditions persisting deeper within the sapropel sediment even after bottom-water conditions have ameliorated to the point of supporting low-oxygen-adapted polychaetes. The nematodes thus burrow downwards and pelletize deeper portions of the sediment than is possible for the polychaetes. Although it is uncertain whether bioturbation and ingestion of the upper sapropel is mainly syndepositional or postdepositional, it is clear that the nematodes interpreted to have fragmented OM laminae and produced type A pellets are better adapted to low-oxygen, sulfidic conditions than even low-oxygen-adapted polychaetes interpreted to have produced type B pellets. Importantly, laminae fragmentation and pelletization by the meiofauna pre-dates emplacement of macroscopic indicators of bioturbation such as Chondrites trace fossils, even though Chondrites is indicative of oxygen-depleted conditions in its own right [46] , [47] . Sediment reworking in some sapropel intervals can be entirely attributed to meiofauna, as macrofaunal trace fossils are absent ( Fig. 2 ). Thus, high-resolution imaging of these Pliocene sapropels shows, for the first time, that comprehensive meiofaunal reworking of organically enriched ancient sediments can occur under low-oxygen, sulfidic conditions prohibitive of macrofaunal metazoan life, consistent with studies of modern sediments showing the ubiquity and dominance of a meiofaunal ‘thiobios’ in equivalent environments [10] . These data does not quantify the changes in organic carbon between ingested and uningested sediment, but studies of modern sediments show that meiofaunal activity exerts an important influence on sediment biogeochemistry, including increased mineralization of sedimentary OM [14] , [15] , [16] . Independent of a direct digestive or enzymatic influence, the extent of meiofaunal burrowing observed in the sapropels implies increased pore-water exchange and solute diffusion relative to undisturbed laminated intervals [16] , [20] . There are no documented examples of comprehensive meiofaunal reworking of marine sediments in the geologic record [22] , [23] , [48] , yet intervals featuring abundant, in situ benthic meiofaunal faecal pellets and fragmented OM laminae are present not only in the Site 969 Pliocene sapropels discussed previously; we also observed these same features in time-equivalent sapropels from the geographically widely-spaced, Eastern Mediterranean ODP Sites 964 and 967 ( Fig. 3e,f ). This raises the question, how common is meiofaunal reworking of sediments under low-oxygen conditions that are prohibitive to macrofauna? While sapropels are commonly used as a model system for anoxic preservation of OM, are they also generally representative of meiofaunal modification that has as yet gone unnoticed in other fine-grained, high-TOC sediments from low-oxygen environments? As noted earlier, although benthic faunal diversity is limited in modern severely dysoxic, sulfidic settings, absolute meiofaunal numbers are not [10] . The common presence of meiofauna in modern oxygen-depleted and sulfidic sediments suggests their presence and influence in ancient sediments is also likely, but may have gone largely unnoticed because of the challenges in detecting their traces. The compositional contrast in BSE images is related to the higher backscatter coefficients of high average atomic number materials such as quartz or carbonate grains, which appear brighter, relative to low average atomic number materials such as OM or carbon-based resin, which appear darker. Identification of fragmented OM laminae and meiofaunal faecal pellets in this study was facilitated by the enrichment of OM in laminae and faecal pellets relative to the OM-lean mineral matrix. We were able to preserve this favourable compositional contrast by utilizing Ar ion milling rather than mechanical polishing before imaging, avoiding the need for resin impregnation that is otherwise required to stabilize poorly consolidate sediments and which would have resulted in substantially reduced BSE contrast between the porous inorganic matrix and OM-rich faecal pellets and laminae fragments. We anticipate that poor compositional or lithological contrast between meiobenthic trace fossils and the sediment matrix is characteristic of many sedimentary deposits, making the routine identification of meiobenthic influence using either conventional light or electron microscopy unlikely. Contrast due to varying compaction or grain orientation is often insufficient to recognize even macrofaunal trace fossils [22] and this is likely to be exacerbated for small, subtle meiofaunal traces, particularly after blurring due to sediment compaction, burial and lithification. In addition, limited vertical mixing by the meiobenthos does not juxtapose contrasting lithologies as does macrofaunal burrowing. Sapropels are utilized as analogues for the widespread, high-TOC black shales that characterize the Palaeozoic and Mesozoic Oceanic Anoxic Events [28] , [29] . Sapropel intervals are relatively thin (1–10 s of cm) compared with many of the Mesozoic black shales (10 s of cm to 10 s of m), and meiofaunal pellets are restricted to the top 3–4 cm of each sapropel due to less severe bottom or pore-water conditions in this upper interval. However, recent work shows that Palaeozoic and Mesozoic black shales are highly heterogeneous at small scales [49] with episodic variation in oxygenation [50] , [51] , so that sulfidic/anoxic intervals are commonly punctuated by dysoxic intervals capable of intermittently supporting benthic foraminifera and even macrofauna such as inoceramids [52] , [53] . Rather than being restricted to the top few centimetres of thick black shale units, sediment reworking by the meiofaunal thiobios could therefore potentially affect a significant proportion of black shales. A further consideration must be the likelihood that meiofaunal bioturbation and homogenization of the sediment is erroneously attributed to later macrofaunal burrowing. In our study, the primary bioturbators in the upper 3–4 cm of the sapropel are undoubtedly the meiofauna, which produce partially laminated to homogeneous intervals that have not previously been recognized as bioturbated because they lack other macroscopically evident indicators of mixing or trace fossils. However, where these meiofaunally reworked intervals are subsequently altered by trace fossil-producing macrofauna, standard ichnological interpretation would incorrectly ascribe the degree of sediment mixing/bioturbation to the benthic macrofauna and also infer that the first metazoan reworking of the sediment occurred under more oxygenated conditions than is required by the meiofaunal thiobios. Thus, the lack of readily observable traces of meiofaunal activity and low familiarity with meiofaunal effects has likely resulted in the attribution of sediment mixing to macrofauna in settings where meiofauna were dominant. This may also be the case in intervals that lack clear evidence for macrofaunal bioturbation. For example, incompletely laminated or homogeneous intervals are commonly interbedded with laminated sediments at a cm to 10 s of cm scale [54] . They are enigmatic as they often lack obvious macrofaunal trace fossils, but since these homogeneous intervals are sometimes transitional to laminated and macroscopically bioturbated intervals, they are generally interpreted to be of macrofaunal origin, produced under bottom waters sufficiently different from the laminated intervals to permit comprehensive macrofaunal bioturbation, but without preservation of trace fossils [54] . Alternatively, they are interpreted as the products of mass flows and sediment liquefaction, or simply a lack of sediment compositional change to define laminae [55] . On the basis of our evidence for meiofaunal homogenization of previously laminated sediments, we would argue that a previously unrecognized meiofaunal origin is equally plausible for these intervals. Finally, recent molecular-clock-based estimates suggest that nematodes arose in the late Neoproterozoic [56] , [57] , potentially as early as the latest Cryogenian. Together with the low-oxygen conditions widely believed to characterize this time in the Earth history, this implies that meiofaunal bioturbation has the potential to explain the occurrence of homogeneous intervals in late Neoproterozoic sediments deposited before the first evidence for bioturbating macrofaunal metazoans at 555 mya [58] , [59] . An investigation of OM-rich, homogeneous or partially laminated Ediacaran mudrocks using our methods may help clarify the extent to which the seemingly abrupt appearance of macrofaunal bilaterians in the fossil record [57] is linked to the prior evolution of cryptic bilaterians of meiofaunal size [27] . Meiofauna have an ecologically and biogeochemically important role in modern marine sediments, but their impact on the sedimentary record remains unknown. Employing an Ar-ion polishing BSE imaging approach, we show extensive meiofaunal reworking and pelletization of the upper 3–4 cm of Pliocene sapropels, a classical anoxic facies, at three geographically widely spaced locations across the Mediterranean. Meiofaunal reworking producing partially laminated to homogeneous sediments pre-dated macrofaunal bioturbation that emplaced macroscopic trace fossils, and occurred under oxygen-depleted and possibly sulfidic conditions that inhibited macrofaunal activity. The dominance of nematodes among the metazoan meiofauna in modern low-oxygen settings, their size and ecology suggests that nematodes are likely responsible for the majority of meiofaunal bioturbation and pelletization of sapropels. Our findings raise the possibility that reworking of high-TOC sediments under oxygen-depleted conditions may have been commonplace in the past. We attribute the lack of previous reports of meiofaunal trace fossils to the absence of a suitable approach for the identification of these cryptic traces, the lack of contrast between lithologies on the small scale of these traces, and the ease with which meiofaunal burrowing can be masked from casual visual observation by later macrofaunal burrowing. We hypothesize that meiofaunal reworking is common in Phanerozoic black shales, where bottom-water or pore-water conditions would rarely have completely inhibited the meiofaunal ‘thiobios’, and we further predict that meiofaunal traces will be most readily identified in high-TOC sediments where alternating OM-rich and OM-lean laminae provide favourable contrast. Late Neoproterozoic OM-rich mudrocks represent a particularly important interval in which to search for similar meiofaunal traces to test predictions of pre-macrofaunal animal history. Ion polishing and electron microscopy We employed scanning electron microscope BSEI (FEI Quanta 450 with energy dispersive X-ray analyser) to image sediment fabric and OM morphology, perpendicular to bedding. Before imaging, samples were oven-dried for 48 h at 60 °C, gently dry-ground until flat, cleaned with compressed nitrogen, ion milled until polished (Fischione 1060 Ar Ion Mill system) and coated with 5 nm Pt. Bulk sample characterization Subsamples for bulk analysis were ground in an agate mortar and pestle. Total carbon was determined with a Perkin Elmer 2400 Series II CHNS analyser. Inorganic C was determined using the pressure calcimeter method of Sherrod et al . [60] , and is reported here as percent carbonate. Organic C content was calculated by difference (TOC=TC-IC), and is reported on a carbonate-free basis (that is, corrected for carbonate dilution). How to cite this article: Löhr, S. C. et al . Micro-trace fossils reveal pervasive reworking of Pliocene sapropels by low-oxygen-adapted benthic meiofauna. Nat. Commun. 6:6589 doi: 10.1038/ncomms7589 (2015).